A mortise–tenon joint in the transmembrane domain modulates autotransporter assembly into bacterial outer membranes Bacterial autotransporters comprise a 12-stranded membrane-embedded β-barrel domain, which must be folded in a process that entraps segments of an N-terminal passenger domain. This first stage of autotransporter folding determines whether subsequent translocation can deliver the N-terminal domain to its functional form on the bacterial cell surface. Here, paired glycine-aromatic ‘mortise and tenon’ motifs are shown to join neighbouring β-strands in the C-terminal barrel domain, and mutations within these motifs slow the rate and extent of passenger domain translocation to the surface of bacterial cells. In line with this, biophysical studies of the autotransporter Pet show that the conserved residues significantly quicken completion of the folding reaction and promote stability of the autotransporter barrel domain. Comparative genomics demonstrate conservation of glycine-aromatic residue pairings through evolution as a previously unrecognized feature of all autotransporter proteins. Autotransporters are integral membrane proteins that play key roles in bacterial pathogenesis. Most autotransporters have large, β-helical passenger domains that are presented on the extracellular surface of bacterial cells; some of these passenger domains remain attached to the surface to function as adhesins, while others are proteolytically processed and released into the environment as effector proteins [1] , [2] , [3] , [4] . The folding of autotransporters is complex, requiring coordination of three reactions, namely (i) the completion of a 12-stranded carboxy-terminal (C-terminal) β-sheet that will wrap to form a β-barrel, but ensuring that (ii) segments of the amino-terminal (N-terminal) domain are entrapped in the luminal cavity of the C-terminal barrel domain and (iii) the folding of the N-terminal passenger domain into its functional form [5] . How these folding reactions are coordinated is unclear. A range of methods have been used to address the folding state of autotransporters in their transit through the periplasm and initiation of assembly into the outer membrane [5] , [6] , [7] , [8] . Several lines of evidence indicate that a threading reaction enabling the passenger domain to emerge from the β-barrel can be completed after insertion into the outer membrane [8] , [9] , [10] , [11] , [12] . For at least some autotransporters, folding of the passenger domain, from its membrane proximal to distal end, assists the process of translocation through the barrel domain [12] and could be driven in part by the free energy change associated with this sort of vectorial protein folding [9] . But what features of the barrel domain enforce control over these processes to ensure the outcome of the folding and assembly process delivers a functional autotransporter onto the bacterial cell surface? In a cellular context, the β-barrel assembly machinery (the BAM complex) catalyses steps in the assembly of autotransporters as it does for other types of β-barrel proteins [12] , [13] , [14] , [15] . Periplasmic chaperones such as SurA also participate in the folding and insertion stages for autotransporters, as does the translocation and assembly module that spans the outer and inner membrane [14] , [16] , [17] , [18] . At least some of these factors might facilitate or retard aspects of protein folding, to assist an overall coordination of the process. Intrinsic features too must play a role in the regulation of the assembly process. Both functional and sequence-based analysis support this supposition: (i) chimeric autotransporters carrying β-barrel domains from other outer membrane proteins showed that efficient passenger domain translocation depends on the barrel domain of an autotransporter [19] and (ii) genome-wide analysis found sequence profile PF03797 (ref. 20) [20] and discrete motifs [21] in the sequences of autotransporters that have been conserved through evolution. One conserved motif referred to as ‘the β-motif’ [21] , appears to act as targeting sequence recognized by the BAM complex [22] , [23] , [24] , [25] , [26] . A second conserved ‘α-linker motif’ was found to be situated within the lumen of several autotransporter barrel domains for which crystal structures are available [21] . Here, we report on structural analysis demonstrating that two other highly conserved motifs, originally referred to simply as motif-3 and motif-4 (ref. 21) [21] , occur in neighbouring strands of the barrel domain. The sequence motifs reflect a structural arrangement of highly conserved residues facing into the lumen of the barrel domain, which we here refer to as a mortise–tenon join that aligns and locks the two neighbouring β-strands, by analogy to the joinery used in woodworking. We sought to understand why these residues have been conserved through evolution, and what they signify in the mechanism of autotransporter assembly. Using a combination of circular dichroism (CD) and fluorescence spectroscopy, limited proteolysis and thermal titrations we find that these conserved residues assist in the controlled folding of barrel domains to accommodate the luminal segment of polypeptide that is so important for correct assembly of autotransporters in bacterial outer membranes. Two sequence motifs converge as a mortise–tenon structure Through structure-based analysis of the sequence motifs conserved in the barrel domains of autotransporters, we identified a highly conserved aromatic residue adopting a notable rotamer conformation: this residue is usually a tyrosine, always faces the β-barrel lumen, and the rotamer has χ -angles [27] , [28] of ‘+60,90’ leaving the residue positioned over the neighbouring β-strand. In this +60,90 conformation, a tyrosine side-chain is compact, extending only 3 Å out from the luminal surface of the β-barrel. 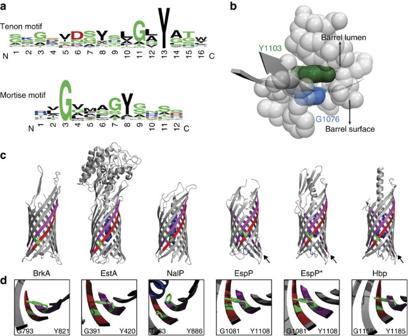Figure 1: A mortise–tenon structure is a highly conserved feature in autotransporters. (a) Sequence Logos describing the tenon motif and mortise motif. Amino acids are coloured according to chemical properties; acidic, red; basic, blue; hydrophilic, green and hydrophobic, black. The height of each letter is proportional to sequence conservation. (b) Representation of the mortise–tenon join in the crystal structure of EspP [pdb code 2QOM]29with Y1103highlighted (dark green). The depicted view through the axis of the barrel, has translucent grey spheres representing the residues surrounding Y1103with G1076shaded light blue, demonstrates that the tyrosine is slotted into the neighbouring residues. Graphic produced in Pymol(The PyMOL Molecular Graphics System, V.r.p., Schrödinger, LLC.). (c) Tenon motif (magenta), mortise motif (red) and, where evident in the crystal structure, the α-linker motif (blue)21were mapped onto the β-barrel domain region of Brk [pdb code 3QQ2]33, EstA [pdb code 3KVN]53, NalP [pdb code 1UYN]54, EspP [pdb code 2QOM]29, ‘precleaved’ EspP*[pdb code 3SLJ]30and Hbp [pdb code 3AEH]31. Arrows indicate position of other strands with statistically significant motifs. The conserved glycine residue and aromatic residue are shown in green. (d) In all β-barrel domain structures other than that of NalP, the conserved aromatic residue in the tenon motif is positioned over the conserved glycine residue in the mortise motif. In the NalP structure, glycine is substituted for threonine. The conserved phenylalanine in the neighbouring strand adopts a −60,90 rotamer, minimizing steric clash with the α-linker segment. Figure 1a shows the conserved tyrosine residue at position 13 in the sequence motif previously referred to as motif-4 (ref. 21) [21] . We now refer to this as the tenon motif ( Fig. 1a ). This tyrosine side-chain locks into a void created by the presence of a highly conserved glycine in position 3 of the neighbouring strand; previously referred to as motif-3 (ref. 21) [21] , we now refer to this as the mortise motif. The nomenclature makes analogy with the mortise–tenon joint used in construction to stabilize adjoining structural elements: Fig. 1b depicts how in the structure of an autotransporter barrel domain, the aromatic residue (dark green) slots into a ‘hole’ created between the backbone of the neighbouring β-strand and the α-helical plug in the barrel lumen. This is made possible only because it is a glycine residue (light blue) at the corresponding position in the neighbouring β-strand ( Fig. 1b ). Crystal structures of the barrel domains of several autotransporters illustrate how the mortise–tenon structure minimizes potential conflicts between the luminal surface of the barrel domain and the ensconced α-linker segment of the autotransporter ( Fig. 1c,d ). Figure 1: A mortise–tenon structure is a highly conserved feature in autotransporters. ( a ) Sequence Logos describing the tenon motif and mortise motif. Amino acids are coloured according to chemical properties; acidic, red; basic, blue; hydrophilic, green and hydrophobic, black. The height of each letter is proportional to sequence conservation. ( b ) Representation of the mortise–tenon join in the crystal structure of EspP [pdb code 2QOM] [29] with Y 1103 highlighted (dark green). The depicted view through the axis of the barrel, has translucent grey spheres representing the residues surrounding Y 1103 with G 1076 shaded light blue, demonstrates that the tyrosine is slotted into the neighbouring residues. Graphic produced in Pymol(The PyMOL Molecular Graphics System, V.r.p., Schrödinger, LLC.). ( c ) Tenon motif (magenta), mortise motif (red) and, where evident in the crystal structure, the α-linker motif (blue) [21] were mapped onto the β-barrel domain region of Brk [pdb code 3QQ2] [33] , EstA [pdb code 3KVN] [53] , NalP [pdb code 1UYN] [54] , EspP [pdb code 2QOM] [29] , ‘precleaved’ EspP*[pdb code 3SLJ] [30] and Hbp [pdb code 3AEH] [31] . Arrows indicate position of other strands with statistically significant motifs. The conserved glycine residue and aromatic residue are shown in green. ( d ) In all β-barrel domain structures other than that of NalP, the conserved aromatic residue in the tenon motif is positioned over the conserved glycine residue in the mortise motif. In the NalP structure, glycine is substituted for threonine. The conserved phenylalanine in the neighbouring strand adopts a −60,90 rotamer, minimizing steric clash with the α-linker segment. Full size image In EspP [29] , [30] [pdb 2QOM] and Hbp [31] [pdb 3AEH] the mortise motif maps to β-strand number 3 of the barrel domain, while a tenon motif maps to β-strand number 4 ( Fig. 1c ). In each case, the aromatic residue in the tenon motif locks in a space created by a conserved glycine in the neighbouring strand ( Fig. 1d ). While the co-conservation of glycine residues in the neighbouring β-strand explains how aromatic residues can be accommodated in the luminal space, the question becomes what functional value might exert the evolutionary pressure to maintain the aromatic residues, given their size and potential conflict with other residues? We used the autotransporter Pet as an experimental model to address this question. Pet was the first identified autotransporter with enterotoxic activity and is a critical virulence factor of enteroaggregative Escherichia coli [32] . The homologous protein from shiga toxin-producing Escherichia coli , called EspP [29] , [30] , has been crystallized thereby providing a means to model the topology of Pet ( Supplementary Fig. 1a ) and three-dimensional structure of Pet ( Supplementary Fig. 1b ). The conserved glycine residue in the mortise motif on β-strand 3 of the Pet β-barrel domain corresponds to residue G 1076 ( Supplementary Fig. 1c ), and this residue was substituted with alanine to create PetG 1076 A. Substitution in the mortise motif perturbs protein stability To directly monitor the folding of the barrel domain, plasmids were engineered for the expression of proteins Pet Δ1–902 and Pet Δ1–902 G 1076 A, encompassing the barrel domain and the 116 residues of the passenger domain immediately N-terminal to the barrel domain ( Supplementary Fig. 1d ). Pet Δ1–902 and the Pet Δ1–902 G 1076 A variant protein were purified in urea and refolded in vitro by rapid dilution of the denaturant in detergent micelles [33] . Pet belongs to the SPATE (serine protease autotransporters of the Enterobacteriaceae ) subfamily of autotransporters, which are characterized by an autocatalytic cleavage of the passenger domain, a reaction that depends on precise positioning of the α-linker segment within the lumen of the correctly folded barrel domain [30] , [31] , [34] . In the cleavage of Pet [32] , the passenger domain is cleaved between asparagine residues N 1018 and N 1019 , and autocatalytic processing of the Pet passenger domain can be used diagnostically as a readout of correct β-barrel folding. The efficiency of the refolding reaction was monitored by the appearance of an ~30 kDa cleavage product from autocatalytic processing of the full-length protein ( Supplementary Fig. 1e ). Cleavage kinetics of Pet Δ1–902 and Pet Δ1–902 G 1076 A barrel domains were obtained by mixing aliquots of the reaction mixture at increasing incubation times with SDS to stop folding ( Fig. 2a , left panel). The unfolded and folded forms were readily separated by SDS–polyacrylamide gel electrophoresis (SDS-PAGE) and quantified by densitometry ( Fig. 2a , right panel), which showed that both Pet Δ1–902 and Pet Δ1–902 G 1076 A refolded with similar efficiencies (46±3% and 35±1%). Cleavage of Pet Δ1–902 followed complex kinetics. A burst amplitude indicated that cleavage commenced within the dead time of the experiment (13±1% of the total amplitude). The burst phase was followed by exponential kinetics that resolved into two phases: the majority of the cleaved protein (22±2%) was cleaved with a faster rate constant of 0.13±0.02 min −1 , whilst a smaller population (11±1% of the amplitude) was cleaved with a significantly slower rate constant of 0.002±0.001 min −1 . Pet Δ1–902 G 1076 A cleavage was slower compared with Pet Δ1–902 with kinetics that were well described by a single exponential phase with a rate constant of 0.004±0.001 min −1 . The rate constant of Pet Δ1–902 G 1076 A cleavage agreed well with the slower rate constant of Pet Δ1–902 cleavage. Two likely interpretations are that folding to the native structure is rate limiting over the slow path, or that the smallest of the Pet Δ1–902 populations and Pet Δ1–902 G 1076 A are folded in an alternative conformation impaired in cleavage compared with the native structure. The latter would suggest that the G 1076 A substitution not merely destabilizes the proteins, but increases the frequency of accessing a non-native conformation. To discriminate whether the delayed cleavage of the Pet Δ1–902 G 1076 A protein was direct or simply concomitant with a delay or change in folding of the β-barrel structure, we monitored protein folding by CD and tryptophan fluorescence spectroscopy and by limited proteolysis. 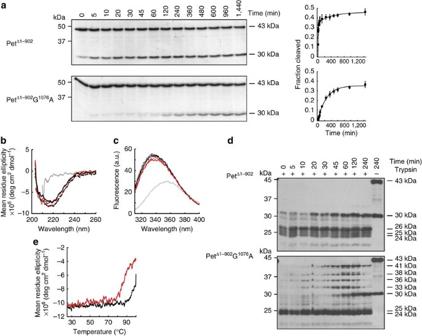Figure 2: Substitution of G1076reduces the cleavage rate, stability and structure of the barrel domain. (a) Folding kinetics of PetΔ1–902and PetΔ1–902G1076A into detergent micelles was monitored by the appearance of the autocatalytically cleaved form (~30 kDa) at the expense of the uncleaved form (~43 kDa) of Pet, analysed by SDS-PAGE and Coomassie blue staining. Densitometry analysis was plotted as a function of time and fitted to exponential functions (right panel). The stated values and error bars correspond to the average and s.d., respectively, of three independent experiments. Far-UV CD (b) and tryptophan fluorescence (c) spectra of unfolded protein (grey), andin vitrofolded and cleaved PetΔ1–902(black) and PetΔ1–902G1076A mutant (red) at t=0 min (full lines) andt=8 h (dashed lines). (d) Folding of PetΔ1–902and PetΔ1–902G1076A monitored by the accumulation of trypsin (20 μg ml−1)-resistant fragments; samples were analysed by SDS-PAGE and immunoblot analysis with anti-barrel domain antibodies. (e) Thermal denaturation ofin vitrofolded, cleaved and purified PetΔ1–902(black) and PetΔ1–902G1076A (red) monitored at 218 nm. Figure 2: Substitution of G 1076 reduces the cleavage rate, stability and structure of the barrel domain. ( a ) Folding kinetics of Pet Δ1–902 and Pet Δ1–902 G 1076 A into detergent micelles was monitored by the appearance of the autocatalytically cleaved form (~30 kDa) at the expense of the uncleaved form (~43 kDa) of Pet, analysed by SDS-PAGE and Coomassie blue staining. Densitometry analysis was plotted as a function of time and fitted to exponential functions (right panel). The stated values and error bars correspond to the average and s.d., respectively, of three independent experiments. Far-UV CD ( b ) and tryptophan fluorescence ( c ) spectra of unfolded protein (grey), and in vitro folded and cleaved Pet Δ1–902 (black) and Pet Δ1–902 G 1076 A mutant (red) at t=0 min (full lines) and t =8 h (dashed lines). ( d ) Folding of Pet Δ1–902 and Pet Δ1–902 G 1076 A monitored by the accumulation of trypsin (20 μg ml −1 )-resistant fragments; samples were analysed by SDS-PAGE and immunoblot analysis with anti-barrel domain antibodies. ( e ) Thermal denaturation of in vitro folded, cleaved and purified Pet Δ1–902 (black) and Pet Δ1–902 G 1076 A (red) monitored at 218 nm. Full size image Far-UV CD spectra of Pet Δ1–902 and Pet Δ1–902 G 1076 A both showed the same characteristic β-signature with minima at 218 nm ( Fig. 2b ), whereas the proteins were completely unfolded in urea. For both variants, the acquisition of secondary structure occurred immediately after rapid dilution of the denaturant with only minor changes observed between the spectra taken at initial and final time points ( Fig. 2b ). Tryptophan fluorescence spectra also indicated a rapid folding of the barrel domain ( Fig. 2c ). The unfolded proteins were characterized by spectra of relatively low intensity and a maximum emission wavelength ( λ max ) around 355 nm, indicating the solvent exposure of the tryptophan residues in this conformation. However, on dilution into detergent micelles, spectra immediately increased in intensity and showed blue-shifted maxima ( Fig. 2c ). The tryptophan residues in Pet Δ1–902 adopted their native state determinants within the dead time of the experiment giving indistinguishable spectra from initial and final samples ( Fig. 2c ). Whilst Pet Δ1–902 G 1076 A also adopted a rapid shift within the experimental dead time, it reproducibly had a diminished fluorescent intensity relative to that in Pet Δ1–902 , even after prolonged incubation ( Fig. 2c ). Importantly, the λ max of the mutant remained red-shifted 5 nm towards higher wavelengths relative to that of the wild-type spectrum (339 nm and 334 nm, respectively), indicating that the tryptophan residues in Pet Δ1–902 G 1076 A do not completely adopt the orientation found in Pet Δ1–902 . Together, these data indicate that both Pet Δ1–902 and Pet Δ1–902 G 1076 A fold rapidly; while perhaps near-native, the conformation of Pet Δ1–902 G 1076 A is at least somewhat distorted. The distorted conformation of Pet Δ1–902 G 1076 A was examined further using limited treatment with trypsin. Titrations of trypsin concentration and digestion times showed that limited digest with 20 μg ml −1 trypsin for 20 min generated discrete sets of proteolytic products. Immediately after the initiation of folding by rapid dilution out of urea, trypsinolysis of Pet Δ1–902 generated two dominant fragments of ~30 kDa and 26 kDa and two other fragments of 25 kDa and 24 kDa ( Fig. 2d ). These fragments provided a kinetic fingerprint by the transient exposure of specific arginine and lysine residues into trypsin-accessible positions during the folding of Pet Δ1–902 . Digestion of Pet Δ1–902 G 1076 A generated a dominant set of 25/24 kDa fragments and a ladder of larger fragments ( Fig. 2d ). The delay in the appearance of a 30-kDa fragment, present at t =0 min for Pet Δ1–902 ( Fig. 2d ), is consistent with the delayed self-cleavage observed for Pet Δ1–902 G 1076 A ( Fig. 2a ). We suggest that the high-molecular weight species between 33 and 41 kDa generated through trypsin digestion represent N-terminal truncated forms of folded Pet Δ1–902 G 1076 A passenger domains that are still attached to the barrel domain ( Fig. 2d ), and that the tryptic fingerprint of the mutant protein is as a result of the folded passenger domain exposing only limited access to trypsin sites. N-terminal sequencing revealed that the 30, 26, 25 and 24 kDa forms of Pet Δ1–902 all start with the cleavage site sequence N 1019 LNKRM ( Supplementary Fig. 1a ). Therefore, the size differences of these fragments result from trypsin cleavages towards the C-terminal end of the barrel domain; trypsin cleavage at arginine and lysine residues in loop L5 and turn T5 correlate well with the size of the fragments ( Supplementary Fig. 1a ). Consistent with this observation, the N-terminal sequence of the 30 kDa form of Pet Δ1–902 G 1076 A is also initiated at N 1019 , evidencing an intact and autocatalytically cleaved barrel domain. However, sequencing of the 25/24 kDa forms of Pet Δ1–902 G 1076 A showed that they initiate from I 1040 within the first transmembrane β-strand: if the barrel domain was folded in a native conformation, this residue would not be accessible to trypsin ( Supplementary Fig. 1a ). Cleavage in Pet Δ1–902 G 1076 A in this position is consistent with the barrel being distorted: taken together, these data show that while the refolded barrel domains are processed autocatalytically between N 1018 and N 1019 in a manner that mimics the in vivo cleavage reaction, the mutant barrel domain tends to adopt a non-native, if near-native, conformation. Many β-barrel proteins, once folded, are resistant to denaturation in SDS at low temperatures, with the folded form showing a faster electrophoretic mobility on SDS-PAGE than the unfolded counterpart [35] , and this ‘heat-modifiability’ is a useful diagnostic tool. The refolded Pet Δ1–902 barrel displayed heat modifiability in SDS at 25 °C, whereas the refolded Pet Δ1–902 G 1076 A barrel appeared completely denatured under these conditions ( Supplementary Fig. 1f ). We complemented these observations with thermal unfolding in CD by monitoring the changes in the β-sheet band at 218 nm ( Fig. 2e ). The data demonstrated that Pet Δ1–902 G 1076 A is less stable than Pet Δ1–902 . Thus, while the Pet Δ1–902 G 1076 A β-barrel domain acquires secondary and tertiary structure, it has a distorted fold, consistent with the observation that the first β-strand is trypsin accessible. We hypothesize that consequent misalignment of the α-linker segment delays the cleavage reaction resulting in inopportune initiation of passenger folding. Translocation of Pet mutants measured in vivo To assess whether the folding defect observed in vitro for PetG 1076 A impacted on autotransporter assembly in vivo , cells harbouring a plasmid for the expression of Pet and PetG 1076 A were induced in the presence of arabinose and, after homogenizing the cells, inner and outer membranes were separated on a discontinuous sucrose gradient. The cleaved Pet and PetG 1076 A barrel domains, detected using antibodies that selectively recognize the barrel domain [15] , migrated in the gradient along with BamA, indicating that Pet and PetG 1076 A had been integrated into the outer membrane ( Fig. 3a ). 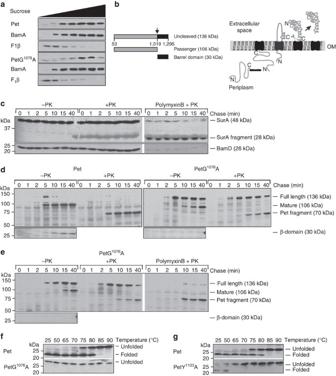Figure 3: Mutation of the mortise motif affects passenger domain translocation and autoproteolytic cleavage. (a) Subcellular location of Pet and PetG1076A after pulse (5 min)-chase (40 min) expression by membrane separation on a discontinuous sucrose gradient. Gradient fractions were analysed by SDS-PAGE and immunoblots stained with anti-Pet barrel domain antibodies. Immunoblotting for the outer membrane protein BamA and the inner membrane F1Fo-ATP synthase F1β subunit served as controls for membrane separation. (b) The domain structure and schematic for biogenesis shows that after synthesis in the cytoplasm Pet is translocated across the inner membrane and processed by the signal peptidase to a 136 kDa polypeptide in the periplasm. Initiation of passenger domain translocation across the outer membrane continues until the N-terminus of the passenger domain traverses the barrel domain pore. Passenger domain folding at the bacterial cell surface results in the α-linker segment being positioned such that autocatalytic cleavage occurs within the lumen of the barrel domain, thereby liberating the 106 kDa passenger domain. (c)E. coliincubated for up to 40 min of a mock ‘chase’ period at 25 °C and then incubated on ice (−PK) or incubated on ice with the addition of 200 μg ml−1proteinase K (+PK) or incubated on ice with the addition of 200 μg ml−1proteinase K and 200 μg ml−1polymyxin B. After addition of Phenylmethanesulfonyl fluoride (see Methods), samples were TCA precipitated and analysed by SDS-PAGE and immunoblotting for SurA or BamD. The intact SurA protein (48 kDa) and a protease-resistant domain of 28 kDa were observed. A shadow corresponding to the migration position of proteinase K (28 kDa) is also observed. BamD is degraded to completion by proteinase K in the presence of Polymyxin B. (d) Pulse-chase Pet and PetG1076A maturation and sensitivity to proteinase K, as indicated (+ or −PK), monitored by SDS-PAGE and immunoblotting with anti-passenger domain antibodies (upper panel) and anti-barrel domain antibodies (lower panel). All samples were TCA precipitated before SDS-PAGE. (e) Pulse-chase PetG1076A maturation as above, but also in the presence of Polymyxin B before addition of proteinase K as indicated (Polymyxin B+PK). (f) Warming to the indicated temperatures of membranes after pulse expression of Pet or PetG1076A, and (g) Warming at the temperatures indicated of membranes following pulse-chase Pet and PetY1103A expression. Samples were analysed by SDS-PAGE and immunoblotting with anti-barrel domain antibodies. Figure 3: Mutation of the mortise motif affects passenger domain translocation and autoproteolytic cleavage. ( a ) Subcellular location of Pet and PetG 1076 A after pulse (5 min)-chase (40 min) expression by membrane separation on a discontinuous sucrose gradient. Gradient fractions were analysed by SDS-PAGE and immunoblots stained with anti-Pet barrel domain antibodies. Immunoblotting for the outer membrane protein BamA and the inner membrane F 1 F o -ATP synthase F 1 β subunit served as controls for membrane separation. ( b ) The domain structure and schematic for biogenesis shows that after synthesis in the cytoplasm Pet is translocated across the inner membrane and processed by the signal peptidase to a 136 kDa polypeptide in the periplasm. Initiation of passenger domain translocation across the outer membrane continues until the N-terminus of the passenger domain traverses the barrel domain pore. Passenger domain folding at the bacterial cell surface results in the α-linker segment being positioned such that autocatalytic cleavage occurs within the lumen of the barrel domain, thereby liberating the 106 kDa passenger domain. ( c ) E. coli incubated for up to 40 min of a mock ‘chase’ period at 25 °C and then incubated on ice (−PK) or incubated on ice with the addition of 200 μg ml −1 proteinase K (+PK) or incubated on ice with the addition of 200 μg ml −1 proteinase K and 200 μg ml −1 polymyxin B. After addition of Phenylmethanesulfonyl fluoride (see Methods), samples were TCA precipitated and analysed by SDS-PAGE and immunoblotting for SurA or BamD. The intact SurA protein (48 kDa) and a protease-resistant domain of 28 kDa were observed. A shadow corresponding to the migration position of proteinase K (28 kDa) is also observed. BamD is degraded to completion by proteinase K in the presence of Polymyxin B. ( d ) Pulse-chase Pet and PetG 1076 A maturation and sensitivity to proteinase K, as indicated (+ or −PK), monitored by SDS-PAGE and immunoblotting with anti-passenger domain antibodies (upper panel) and anti-barrel domain antibodies (lower panel). All samples were TCA precipitated before SDS-PAGE. ( e ) Pulse-chase PetG 1076 A maturation as above, but also in the presence of Polymyxin B before addition of proteinase K as indicated (Polymyxin B+PK). ( f ) Warming to the indicated temperatures of membranes after pulse expression of Pet or PetG 1076 A, and ( g ) Warming at the temperatures indicated of membranes following pulse-chase Pet and PetY 1103 A expression. Samples were analysed by SDS-PAGE and immunoblotting with anti-barrel domain antibodies. Full size image We established a time course assay for the pulse-chase expression of Pet and PetG 1076 A in whole cells, monitored by immunoblot analysis after SDS-PAGE using antibodies that selectively recognize the passenger domain [32] . This provided the means to assess the processing of the secreted form of the ~106 kDa passenger domain and residual ~30 kDa barrel domain, from the uncleaved ~136 kDa protein ( Fig. 3b ). In addition, at each time-point, an aliquot was treated with proteinase K to digest the population of molecules that were surface exposed: preliminary experiments were done to titrate the amount of proteinase K in use, so as to be sufficient to cleave the periplasmic protein SurA and the lipoprotein BamD that are exposed to the periplasm, but only when polymyxin B was also present ( Fig. 3c ); polymyxin B is an antibiotic that selectively permeabilizes the outer membrane [36] , [37] . A time course of pulsed-chase expression of Pet and PetG 1076 A in intact cells demonstrated that Pet processing into distinct passenger domain and barrel domain was underway by 5 min and largely completed by 10 min ( Fig. 3d , left panel, −PK). Proteinase K digestion of Pet was also observed after 5 min, indicating that uncleaved Pet was exposed on the cell surface by this time-point ( Fig. 3d , left panel, +PK). In contrast, the cleavage of PetG 1076 A occurred with much reduced efficiency, with only ~50% processing of the 136 kDa species to the 106 kDa mature species after 40 min ( Fig. 3d , right panel, −PK). The 136 kDa form of PetG 1076 A was only degraded by proteinase K in the presence of polymyxin B, indicating that a substantial part of the protein is exposed to the periplasm ( Fig. 3e ). A 70 kDa passenger domain fragment of PetG 1061 A behaves similarly under these conditions ( Fig. 3e ). To address what appeared to be a decrease in the steady-state level of the barrel domain of PetG 1061 A relative to Pet ( Fig. 3d ), we tested the thermal stability of the barrel lacking the key residues in the mortise and tenon motifs. The cleaved barrel domain of Pet was resistant to SDS denaturation, showing greater electrophoretic mobility (that is, the ~25 kDa form of the protein) in samples heated up to 70 °C and with total denaturation of the β-structure above 85 °C ( Fig. 3f ). In contrast, the PetG 1076 A mutant migrated as completely denatured in SDS at all temperatures. The aromatic residue in the tenon motif also plays a role in barrel domain folding: a PetY 1103 A mutation also resulted in a defect in the thermal stability of the barrel domain, albeit less pronounced ( Fig. 3g ). Either the mortise–tenon structure maintains Pet resistance to SDS, or it is crucial for correct folding of the barrel in vivo , as in vitro . Evolution has selected for mortise–tenon sequences Multiple occurrences of each of these motifs were evident in the evaluation of the autotransporter protein family ( Supplementary Fig. 2 ). This suggests that while motif searches are a useful sequence tool to detect the mortise–tenon structure, the searches underestimate the number of occurrences in each autotransporter sequence. To address whether other glycine residues might be conserved for similar structural reasons, an independent approach was taken using the Position Specific Scoring Matrix generated by the Conserved Domain Database [38] , [39] . This tool uses multiple sequence alignments to calculate and depict the relative frequencies of amino acid residues at each position in the barrel domain of autotransporter sequences ( Supplementary Fig. 3a ). Inspection of the most frequently occurring residues at each position suggested several highly conserved residues including a tryptophan, two tyrosine residues and five glycine residues ( Supplementary Fig. 3b ). On the topology model ( Fig. 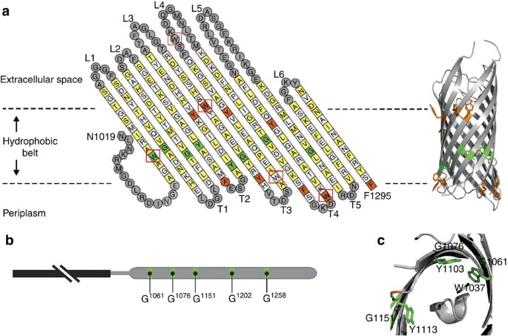Figure 4: Distribution of conserved glycine and aromatic residues around the barrel domain of autotransporters. (a) Topology model of Pet, detailing the location of conserved residues W1037(β-strand 1), G1061(β-strand 2), G1076(β-strand 3), Y1103(β-strand 4), Y1113(β-strand 5), G1151(β-strand 6), G1202(β-strand 8) and G1258(β-strand 10) in green. In the topology diagram, white and yellow squares indicate residues with side chains that point toward the barrel lumen and the lipid bilayer, respectively. Extracellular loops (L1-L6) and periplasmic turns (T1-T5) are labelled. The residues that form the extracellular and periplasmic aromatic girdles are highlighted in orange. These are anticipated to align with the membrane interfaces and therefore define the positioning of the barrel within the plane of the outer membrane55,56. The location of the tryptophan residues used to obtain information on the folding of the barrel domain using the intrinsic fluorescent properties of Pet are boxed: W1037(β-strand 1), W1144(β-strand 6), W1161(β-strand 7), W1180(L4), W1214(β-strand 9). Also shown is a structural model of Pet, with conserved glycine and aromatic residues shown in green, and the residues that form the extracellular and periplasmic aromatic girdles highlighted in orange. (b) Schematic view of the positions of the residues subjected to mutagenesis inFig. 5. (c) A cross-section view through the crystal structure of the EspP barrel domain demonstrates that like G1076in the mortise motif, G1061and G1151also have a conserved aromatic residue that adopts an unusual position to bend tightly over them (W1037and Y1113, respectively). 4a ) of Pet, some of these residues map to neighbouring β-strands: strands 1 and 2 (W 1037 and G 1061 ), strands 3 and 4 (G 1076 and Y 1103 ), strands 5 and 6 (Y 1113 and G 1151 ) as summarized in Figure 4b , while the other two conserved residues G 1202 and G 1258 on strands 8 and 10. Collectively, they form a ring positioned between the extracellular and periplasmic aromatic annuli of the β-barrel, but visual inspection of the barrel domain structure revealed G 1061 , G 1076 and G 1151 participate in mortise–tenon structures ( Fig. 4c ). To survey the impact of all conserved glycine residues on Pet biogenesis, we introduced an alanine residue at these positions and induced cells harbouring a plasmid for the expression of Pet, PetG 1061 A, PetG 1151 A, PetG 1202 A and PetG 1258 A in response to the presence of the inducer arabinose. Figure 4: Distribution of conserved glycine and aromatic residues around the barrel domain of autotransporters. ( a ) Topology model of Pet, detailing the location of conserved residues W 1037 (β-strand 1), G 1061 (β-strand 2), G 1076 (β-strand 3), Y 1103 (β-strand 4), Y 1113 (β-strand 5), G 1151 (β-strand 6), G 1202 (β-strand 8) and G 1258 (β-strand 10) in green. In the topology diagram, white and yellow squares indicate residues with side chains that point toward the barrel lumen and the lipid bilayer, respectively. Extracellular loops (L1-L6) and periplasmic turns (T1-T5) are labelled. The residues that form the extracellular and periplasmic aromatic girdles are highlighted in orange. These are anticipated to align with the membrane interfaces and therefore define the positioning of the barrel within the plane of the outer membrane [55] , [56] . The location of the tryptophan residues used to obtain information on the folding of the barrel domain using the intrinsic fluorescent properties of Pet are boxed: W 1037 (β-strand 1), W 1144 (β-strand 6), W 1161 (β-strand 7), W 1180 (L4), W 1214 (β-strand 9). Also shown is a structural model of Pet, with conserved glycine and aromatic residues shown in green, and the residues that form the extracellular and periplasmic aromatic girdles highlighted in orange. ( b ) Schematic view of the positions of the residues subjected to mutagenesis in Fig. 5 . ( c ) A cross-section view through the crystal structure of the EspP barrel domain demonstrates that like G 1076 in the mortise motif, G 1061 and G 1151 also have a conserved aromatic residue that adopts an unusual position to bend tightly over them (W 1037 and Y 1113 , respectively). Full size image There were no obvious differences in the insertion, assembly and cleavage of PetG 1151 A, PetG 1202 A and PetG 1258 A relative to that observed in wild-type Pet ( Fig. 5a ). However, substitution of an alanine residue was more detrimental in PetG 1061 A, with both a delayed arrival at the cell surface and a slower processing into mature passenger and β-barrel domain ( Fig. 5a ). Like the PetG 1076 A mutant, the PetG 1061 A protein appears to be exposed on the outer surface of the outer membrane, since in the absence of polymyxin B, the mature 106 kDa form of PetG 1061 A is proteinase K sensitive ( Fig. 5b ). In contrast, the 136 kDa form of PetG 1061 A was only degraded by proteinase K in the presence of polymyxin B, indicating that a substantial part of that form of the protein is exposed to the periplasm ( Fig. 5b ). PetG 1151 A, PetG 1202 A and PetG 1258 A were only marginally destabilized relative to wild-type Pet ( Fig. 5c ). However, as was the case for PetG 1076 A, the PetG 1061 A mutant protein is denatured in SDS at all temperatures ( Fig. 5c ), demonstrating that interfering with either of these conserved glycine residues impacts significantly on the folding pathway for the autotransporter. 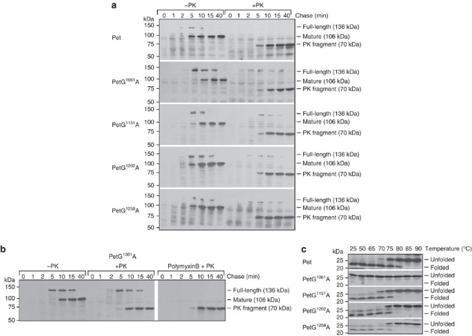Figure 5: Like G1076the conserved G1061impacts on Pet translocation and barrel domain stability. (a) Pulse-chase maturation and proteinase K sensitivity, as indicated (+ or −PK), of Pet, PetG1061A, PetG1151A, PetG1202A or PetG1258A. (b) Pulse-chase maturation and proteinase K sensitivity of PetG1061A, as indicated (+ or −PK, or Polymyxin B+PK). Samples were TCA precipitated (inaandb) before analysis by SDS-PAGE and immunoblotting with anti-passenger domain antibodies. (c) Warming to the indicated temperatures of membranes after pulse expression of Pet, PetG1061A, PetG1151A, PetG1202A or PetG1258A. Samples were analysed by SDS-PAGE and immunoblotting with anti-barrel domain antibodies. Figure 5: Like G 1076 the conserved G 1061 impacts on Pet translocation and barrel domain stability. ( a ) Pulse-chase maturation and proteinase K sensitivity, as indicated (+ or −PK), of Pet, PetG 1061 A, PetG 1151 A, PetG 1202 A or PetG 1258 A. ( b ) Pulse-chase maturation and proteinase K sensitivity of PetG 1061 A, as indicated (+ or −PK, or Polymyxin B+PK). Samples were TCA precipitated (in a and b ) before analysis by SDS-PAGE and immunoblotting with anti-passenger domain antibodies. ( c ) Warming to the indicated temperatures of membranes after pulse expression of Pet, PetG 1061 A, PetG 1151 A, PetG 1202 A or PetG 1258 A. Samples were analysed by SDS-PAGE and immunoblotting with anti-barrel domain antibodies. Full size image Recently, six sequence motifs were identified which, as a group, can be used to detect and classify autotransporters from genome sequence data [21] . The functional significance of two of these motifs has now been revealed: they represent conserved sequence signatures that enable a neighbouring pair of β-strands to anneal with each other such that the large side-chain of an aromatic residue in one strand (corresponding to the tenon motif) intercalates into the space made available by the specific positioning of a glycine residue in the neighbouring strand (in the mortise motif). We have also discovered that this joint between neighbouring β-strands can also occur in positions which are not readily recognized by motif analysis, that is, only some of these mortise–tenon structures can be predicted with statistical significance. The Position Specific Scoring Matrix screen of autotransporter sequences in concert with visual inspection of the available crystal structures shows this common structural joinery between neighbouring strands is a prevalent feature in autotransporters. Conceptually, the mortise–tenon structures can explain the molecular basis for mutant phenotypes seen in two previous studies. The autotransporter Hbp (also known as Tsh) has several conserved sequences [40] and mutations in these diminish its assembly in E. coli . In one case, HbpG 1158 Y, a specific defect was characterized by accumulation of an unprocessed form of Hbp in the periplasm [41] . G 1158 sits in a mortise motif in the Hbp sequence, and analysis of the crystal structure of Hbp shows that the neighbouring β-strand carries a conserved aromatic residue (Y 1185 ), where HbpG 1158 and HbpY 1185 are the equivalent of PetG 1076 and PetY 1103 ( Supplementary Fig. 1c ). Conversely, mutational analyses of EspP show delayed passenger domain translocation in the mutant proteins EspPG 1066 A and EspPG 1081 D, that did not affect interactions with the periplasmic chaperone Skp nor the BAM complex [42] . It was concluded that these mutations affect the insertion of the EspP barrel domain into the plane of the outer membrane [42] . Analysis of the crystal structure of EspP shows that these mutations, EspPG 1066 A and EspPG 1081 D, would each affect a mortise–tenon structure ( Supplementary Fig. 1c ). Taken together with the delay of PetG 1076 A to become surface exposed in intact E. coli and its slowed rate of autocatalytic processing on folding in vitro , we conclude that correctly formed interstrand joins are required in order to efficiently incorporate the passenger domain, thereby promoting efficient translocation through the lumen of the barrel domain. Our results indicate that mortise–tenon structures promote efficient folding of an autotransporter, providing a rationale for the selection of these structures through the course of evolution: the conserved residues would assist in correctly registering neighbouring β-strand hairpins during the folding reaction. We hypothesize that their removal increases the ruggedness of the folding landscape, promoting misfolding as evidenced by the trypsin susceptibility of the first β-strand in a population of the molecules of the PetG 1076 A protein, and the decreased thermal stability of the PetG 1076 A and the PetY 1103 A proteins. Related to this, a mortise–tenon structure allows, and is completed by, correct packing of the α-linker segment in the lumen of the autotransporter barrel domain, thereby further stabilizing the β-barrel structure [30] , [31] , [43] . Regulation over the folding reaction is essential to obtain a functional autotransporter. Secretion of autotransporter passenger domains across the outer membrane requires that, ultimately, the polypeptide has extended through an aqueous channel that is formed by the barrel domain [5] . Thus, unlike other β-barrel proteins, the folding of an autotransporter barrel domain needs to proceed in a controlled fashion that also allows positioning of a segment of the passenger domain within the barrel domain lumen: in the correct structural context, and before the first and last β-strands anneal with each other to close the barrel domain. Cellular factors including the BAM and the translocation and assembly module have been identified which can act in trans to facilitate or retard aspects of protein folding, presumably to assist in coordinating the process as it occurs in the outer membrane [12] , [13] , [14] , [15] . It has been postulated that in order to facilitate positioning and translocation of the passenger domain through the lumen in the barrel domain, non-native ‘barrel-like’ conformations might be adopted within the outer membrane: perhaps including an additional β-strand, or a more rounded conformation, or an incomplete annealing of neigbouring β-strands [44] . There are distinct views on whether the appropriate segment of polypeptide first positioned in the barrel would (i) encompass part of the α-linker segment or (ii) be a more distal region of the passenger domain, and only after considerable translocation would the α-linker segment take up its correct position. There is some experimental support for each view [10] , [12] , [45] , but in any of these models, control over this complex folding process holds the key to the success in initiating autotransporter assembly. Our findings indicate that the key residues facing into the barrel lumen have been under positive selective pressure through the course of evolution to achieve exactly that. In summary, the mortise–tenon interaction favors the alignment of β-strands and incorporation of the passenger domain to improve translocation kinetics in vivo . Experiments with the purified proteins refolded in vitro verify that the conserved features in these neighbouring strands have a direct effect on protein stability. These aspects of structure would assist folding of the β-strands into a β-sheet, and coordinate this with the inward folding of the segment of passenger domain that first occupies the barrel lumen, ultimately creating a device that can efficiently promote passenger domain translocation onto the bacterial cell surface. The significance of the mortise–tenon structure is evident in the prevalence with which it has been selected for through evolution as a fundamental feature of autotransporters. Reagents and bacterial strains Unless otherwise stated, bacteria were grown at 37 °C in Luria-Bertani broth and where necessary, the growth medium was supplemented with 100 μg ml −1 ampicillin, 0.2% (v/v) D -glucose, 0.02% (v/v) L -arabinose, or 0.5 mM isopropylthio-β-galactoside. Details of the E. coli strains (TOP10 and BL21 (DE3)) and plasmids used in this study are presented in Table 1 , and primers used for plasmid construction are presented in Table 2 . Table 1 Strains and plasmids used in this study. Full size table Table 2 Primers used in this study. Full size table Plasmid construction pBADPet has been described previously [46] . To construct pBADPetG 1061 A, pBADPetG 1076 A, pBADPetG 1151 A and pBADPetY 1103 A, megaprimer PCR was performed as described previously [47] , [48] with some variation. Briefly, all round 1 PCRs were performed on 500 ng of template DNA (pBADPet) with 1 μg of the appropriate mutagenesis primer always in combination with 1 μg of primer AatIIRv per 100 μl reaction mixture. Round 1 PCRs were then purified to remove residual primers from the megaprimer synthesized in this first round of amplification. Round 2 PCRs were performed with 4 μg of megaprimer and 1 μg of primer EagIFw on 500 ng of template DNA (pBADPet) per 100 μl reaction mixture. Round 2 amplicons and target vector (pBADPet) were then digested with EagI and AatII and ligated. Construct pBADPetG 1202 A and pBADPetG 1258 A were generated as described above with the exception that round 1 PCRs were performed with the appropriate mutagenesis primer and primers EcoRIRv and HindIIIRv, respectively. Round 2 PCRs ensued using primers EagIFw and AatIIFw, respectively and the subsequent amplicons and target vector (pBADPet) were then digested with EagI and EcoRI (pBADPetG 1202 A) and, AatII and HindIII (pBADPetG 1258 A), and ligated. To construct pETPet Δ1–902 , the Pet barrel domain and the last 116 residues of the Pet passenger domain were amplified using 500 ng of template DNA (pBADPet) with 1 μg each of primers NdeIPetFw and XhoIPetRv. The subsequent amplicon and target vector (pET-22b+) were then digested with NdeI and XhoI, and ligated for an in frame C-terminal hexahistidine-tag fusion. pETPet Δ1–902 G 1076 A was generated as above with the exception that PCRs were amplified using pBADPetG 1076 A template DNA. Pulse-chase protein expression assay The pBAD expression system [49] was used to produce protein. Bacterial cultures grown to mid-log phase in glucose to repress Pet synthesis were harvested (2,500 × g , 5 min, 4 °C), and then Pet expression was induced with arabinose for 5 min (pulse). Bacterial cells were recovered and resuspended in media containing glucose at 25 °C to ‘chase’ the protein produced during the ‘pulse’ phase of the experiment through the translocation pathway. Following the pulse-chase assay, four 1 ml aliquots were removed from each culture. The first aliquot was added to a tube containing a 10% (w/v) final concentration of trichloroacetic acid (TCA) and placed on ice. The second aliquot was treated with 200 μg ml −1 proteinase K for 20 min on ice to digest Pet exposed on the cell surface and the third aliquot was treated with 200 μg ml −1 polymyxin B for 10 min on ice as previously described [36] , [37] before proteinase K treatment. Phenylmethanesulfonyl fluoride (PMSF) at 2 mM final concentration was used to stop the protease reaction before TCA precipitation. All TCA-precipitated samples were washed with acetone, dried and resuspended in 100 μl of SDS-PAGE loading buffer per 1 OD600 units of cells (fourth aliquot). Samples were analysed by SDS-PAGE on 3–14% gradient gels followed by immunoblotting using anti-passenger domain and anti-barrel domain antibodies both used at a 1:5,000 dilution. These antibodies have been described and validated previously [15] , [32] . Briefly, to raise anti-barrel domain antibodies, the sequence corresponding to the Pet barrel domain was cloned into the pMAL-c2X expression vector, and the resulting maltose-binding protein-Pet barrel domain fusion was purified in accordance with the manufacturer’s instructions. For anti-passenger domain antibodies, the Pet passenger domain was isolated from culture supernatant of enteroaggregative E. coli O42 and purified using DEAE-cellulose and Sephadex columns, before immunization of rabbits and subsequent harvesting of serum. Subcellular fractionation and heat modifiability assays After pulse-chase protein expression, cells were harvested and prepared for sucrose density gradient centrifugation as described previously [50] . In heat modifiability experiments, 40 μg of total membranes were mixed with SDS-PAGE loading buffer and then heated at temperatures between 25 °C and 90 °C. All samples were resolved by SDS-PAGE on 3–14% gradient gels and subjected to immunoblotting using anti-barrel domain antibodies as described above. Protein expression and purification Protein expression and refolding followed previously described methodology [33] . Briefly, E. coli BL21 (DE3) cells transformed with pETPet Δ1–902 and pETPet Δ1–902 G 1076 A were harvested after induction with 0.5 mM isopropylthio-β-galactoside, from which inclusion bodies were isolated for protein purification in 8 M urea. Pet Δ1–902 and Pet Δ1–902 G 1076 A were then refolded from the urea extracts by rapid 10-fold dilution into 0.5% (w/v) lauryldimethylamine-oxide detergent micelles at 37 °C. After affinity purification using Ni-NTA resin, further purification by gel filtration chromatography (Superdex s200-10/300, GE HealthCare) resulted in purification of the folded ~30 kDa form. For N-terminal amino acid sequencing of the trypsin treated Pet Δ1–902 and Pet Δ1–902 G 1076 A barrel domain fragments, proteins were first separated by 12% SDS-PAGE and blotted onto a polyvinylidene difluoride sequencing-grade membrane. After blotting, proteins were visualized by staining with Coomassie brilliant blue (R-250), and the appropriate bands were excised and sequenced by automated Edman degradation at the Biomedical Proteomics Facility (Monash University) [51] . Biophysical analysis of protein structure Folding kinetics of the Pet Δ1–902 and Pet Δ1–902 G 1076 A barrel domains were measured after folding was initiated by rapid dilution of the unfolded proteins into detergent micelles at 37 °C as described above [33] . Small aliquots of the reaction mixture were removed and quenched with SDS loading buffer (final concentration of SDS: 1% w/v) at the time points indicated, and immediately heated at 100 °C. The unfolded and folded forms were separated by SDS-12% PAGE and band intensities were integrated by densitometry to determine the fraction cleaved for each time point. The Pet Δ1–902 data fitted to a double exponential equation (y= A burst+ A fast*(1−exp(− k fast* t )+ A slow*(1−exp(− k slow* t )) and the Pet Δ1–902 G 1076 A data to a single exponential equation (y= A slow*(1−exp(− k slow* t )) where y is the fraction cleaved at a given time ( t ), A is the amplitude and k is the rate constant. The stated values and error bars correspond to the average and s.d., respectively, of three independent experiments. Kinetics of trypsin cleavage profiles during Pet Δ1–902 and Pet Δ1–902 G 1076 A folding were initiated as described above. Limited treatment with trypsin was performed as described previously [52] . Aliquots of the reaction mixture were removed and treated with trypsin (20 μg ml −1 ) for 20 min on ice at the time points indicated. Following trypsin treatment, digestions were quenched with 2 mM PMSF, SDS loading buffer was added to each sample and the resulting trypsin fragments were separated by SDS-PAGE and subjected to immunoblotting using anti-barrel domain antibodies as described above. Far-UV CD spectra were collected from 190 to 260 nm using a Jasco J-815 spectropolarimeter. Folding of Pet Δ1–902 and Pet Δ1–902 G 1076 A barrel domains was initiated as described above and monitored at 37 °C for 8 h in a 1-mm cuvette after removing aliquots of the reaction mixture containing 0.1 mg ml −1 of protein. The bandwidth was set to 1.0 nm, integration time 1 s, scanning speed 20 nm/min, three scans were averaged, and the spectrum was subtracted for buffer contribution. For thermal denaturation measurements, the change in CD signal at 218 nm was measured as a function of temperature from 25–100 °C at a temperature change of 1 °C min −1 . In both cases, the measured CD spectra were normalized to the mean residue molar ellipticity. Thermal unfolding was irreversible. A Varian Cary Eclipse fluorimeter was used for all fluorescence measurements. Samples containing 0.01 mg ml −1 of protein were collected at t =0 min and t =8 h after folding of Pet Δ1–902 and Pet Δ1–902 G 1076 A barrel domains was initiated as described above, and measured at 25 °C, in a 1-cm cuvette. The emission spectra were collected between 300–400 nm on excitation of tryptophan at 295 nm, with an integration time of 0.1 s, a slit width of 5 nm and an increment of 1.0 nm. Three scans were averaged and the spectra were corrected for buffer contribution. How to cite this article: Leyton, D. L. et al. A mortise–tenon joint in the transmembrane domain modulates autotransporter assembly into bacterial outer membranes. Nat. Commun. 5:4239 doi: 10.1038/ncomms5239 (2014).